Proteasomal degradation of Nck1 but not Nck2 regulates RhoA activation and actin dynamics The ubiquitously expressed adapter proteins Nck1/2 interact with a multitude of effector molecules to regulate diverse cellular functions including cytoskeletal dynamics. Here we show that Nck1, but not Nck2, is a substrate of c-Cbl-mediated ubiquitination. We uncover lysine 178 in Nck1 as the evolutionarily conserved ubiquitin acceptor site. We previously reported that synaptopodin, a proline-rich actin-binding protein, induces stress fibres by blocking the Smurf1-mediated ubiquitination of RhoA. We now find that synaptopodin competes with c-Cbl for binding to Nck1, which prevents the ubiquitination of Nck1 by c-Cbl. Gene silencing of c-Cbl restores Nck1 protein abundance and stress fibres in synaptopodin knockdown cells. Similarly, expression of c-Cbl-resistant Nck1(K178R) or Nck2 containing the SH3 domain 2 of Nck1 restores stress fibres in synaptopodin-depleted podocytes through activation of RhoA signalling. These findings reveal proteasomal regulation as a key factor in the distinct and non-redundant effects of Nck on RhoA-mediated actin dynamics. The Nck protein family consists of two members, Nck1 (Nckα) and Nck2 (Nckβ), which contain three SH3 domains and a single SH2 domain. Nck1 and Nck2 share 68% amino-acid identity [1] . Ncks are widely expressed adapter proteins that can bind to phosphotyrosine residues on kinases via their SH2 domain or recruit proline-rich proteins via their SH3 domains [2] . Ncks can mediate signalling from cell surface receptors to the actin cytoskeleton by stimulating N-WASP-Arp2/3-induced actin nucleation [3] , [4] or by activating Pak1 (ref. 5 ). Pericyte-like podocytes, whose cytoskeletal integrity is essential for proper filter function [6] , serve as an excellent model system for the study of actin dynamics [7] . In podocytes, Nck proteins stabilize the actin cytoskeleton by regulating the phosphorylation of the slit diaphragm protein nephrin, and podocyte Nck function is essential for the development and maintenance of the glomerular filtration barrier [8] , [9] , [10] . Synaptopodin is a proline-rich actin-binding protein strongly expressed in highly dynamic cell compartments such as dendritic spines in the brain and podocyte foot processes in the kidney [7] , [11] . Gene silencing of synaptopodin in podocytes causes the loss of stress fibres and the concomitant development of aberrant, non-polarized, filopodia [12] , [13] . Synaptopodin is a positive regulator of RhoA and a negative regulator of Cdc42 signalling [13] , [14] . Synaptopodin can directly bind to RhoA and induces stress fibres by competitively blocking the Smurf1-mediated ubiquitination of RhoA, thereby preventing the targeting of RhoA for proteasomal degradation [13] , [15] . Here we identify a mechanism for the co-regulation of RhoA signalling by Nck and synaptopodin. We show that, in addition to inhibiting the Smurf1-mediated ubiquitination and subsequent proteasomal degradation of RhoA by blocking the binding of Smurf1 to RhoA [13] , synaptopodin also prevents the targeting of a pool of Nck1 for proteasomal degradation by blocking the binding of c-Cbl to Nck1, which in turn increases RhoA activity and stress fibre formation. We further show that the second SH3 domain of Nck1 is essential for the observed effects of Nck1 on stress fibre formation. Taken together, these results unveil the c-Cbl-mediated ubiquitination of Nck1 as an additional layer of the ever-growing signalling machinery that controls Rho proteins and actin dynamics. Nck1/2 bind to synaptopodin Synaptopodin exists in the following three isoforms ( Fig. 1a ): renal synpo-long (903AA), neuronal synpo-short (685 AA) and Synpo-T, which is identical to the C-terminal 181 AA of Synpo-long and serves as a backup of Synpo-long during kidney development in synaptopodin null mice [12] . Synaptopodin can bind to SH3 domain containing proteins, including CD2AP [16] and IRSp53 (ref. 14 ). Here we asked whether synaptopodin could also interact with the SH3 domain containing Nck proteins. In support of this, in heterologous co-immunoprecipitation (Co-IP) experiments in co-transfected HEK293 cells, we found that both GFP (green-fluorescent protein)-Nck1 and GFP-Nck2 could bind to FLAG-tagged Synpo-long, Synpo-short or Synpo-T isoforms [13] ( Fig. 1b ). The interaction of GFP-Nck1 and GFP-Nck2 with FLAG-N-WASP [3] served as a positive control. No interaction of synaptopodin or N-WASP was found with GFP-sui serving as a negative control ( Fig. 1b ), thereby confirming the specificity of the interaction. The interaction between synaptopodin and Nck was further examined by endogenous Co-IP studies using anti-Nck antibodies that showed relative selectivity and specificity for Nck1 and Nck2, respectively, in western blot analysis of whole-cell lysates of HEK292 cells transfected with GFP-Nck1 or GFP-Nck2 ( Fig. 1c ). In protein extracts from isolated glomeruli, both anti-Nck1 or anti-Nck2 antibodies co-precipitated synaptopodin ( Fig. 1d ). Conversely, anti-synaptopodin antibody precipitated synaptopodin and co-precipitated Nck1 and Nck2 ( Fig. 1d ). To test whether Nck can directly bind to synaptopodin, we incubated purified GST-Nck1, GST-Nck2 or GST with purified FLAG-Synpo-long, FLAG-Synpo-short, or FLAG-Synpo-T and found a specific interaction of all three synaptopodin isoforms with GST-Nck1 and GST-Nck2 but not the GST control ( Fig. 1e ). We also detected direct binding of GST-Nck1 and GST-Nck2 to FLAG-N-WASP serving as positive control ( Fig. 1e ). Thus, as there is no sequence overlap between Synpo-S and Synpo-T [12] , at least two distinct Nck-binding interfaces exist, one in Synpo-S and one in Synpo-T. 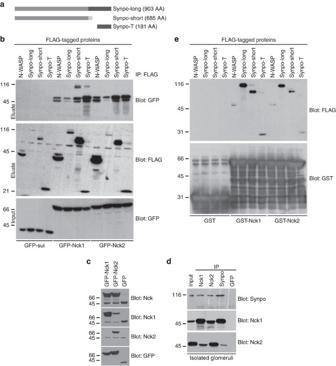Figure 1: Nck directly binds to synaptopodin. (a) Schematic of synaptopodin isoforms. (b) GFP-Nck1 and GFP-Nck2 co-precipitate with FLAG-Synpo-long, FLAG-Synpo-short and FLAG-Synpo-T from co-transfected HEK293 cells. No interaction is found with GFP-sui serving as negative control. The interaction between FLAG-N-WASP and GFP-Nck1/2 serves as positive control. (c) Western blot analysis of Nck antibody specificity in HEK293 cells transfected with GFP-Nck1, GFP-Nck2 or GFP. (d) Endogenous Co-IP shows that Nck1 and Nck2 interact with synaptopodin in isolated mouse glomeruli. IP with anti-GFP (control) serves as negative control. IP: immunoprecipitation. (e) Direct binding of purified FLAG-Synpo to purified GST-Nck1 and GST-Nck2 but not the GST control. The interaction between purified FLAG-N-WASP and GST-Nck1/2 serves as positive control. Molecular weight markers are in kDa. Figure 1: Nck directly binds to synaptopodin. ( a ) Schematic of synaptopodin isoforms. ( b ) GFP-Nck1 and GFP-Nck2 co-precipitate with FLAG-Synpo-long, FLAG-Synpo-short and FLAG-Synpo-T from co-transfected HEK293 cells. No interaction is found with GFP-sui serving as negative control. The interaction between FLAG-N-WASP and GFP-Nck1/2 serves as positive control. ( c ) Western blot analysis of Nck antibody specificity in HEK293 cells transfected with GFP-Nck1, GFP-Nck2 or GFP. ( d ) Endogenous Co-IP shows that Nck1 and Nck2 interact with synaptopodin in isolated mouse glomeruli. IP with anti-GFP (control) serves as negative control. IP: immunoprecipitation. ( e ) Direct binding of purified FLAG-Synpo to purified GST-Nck1 and GST-Nck2 but not the GST control. The interaction between purified FLAG-N-WASP and GST-Nck1/2 serves as positive control. Molecular weight markers are in kDa. Full size image Synaptopodin stabilizes Nck1 but not Nck2 protein abundance Undifferentiated podocytes lack synaptopodin and display a cortical actin cytoskeleton as well as low levels of RhoA expression [12] , [13] , [17] . In western blots from undifferentiated podocyte lysates, we found low Nck1, but high Nck2 and c-Cbl protein abundance ( Fig. 2a , left). In contrast, differentiated podocytes or differentiated podocytes infected with a non-silencing control short hairpin RNA (shRNA) displayed robust synaptopodin [12] , [13] , [17] and Nck1 protein abundance ( Fig. 2a ; left panels). Gene silencing of synaptopodin led to the downregulation of Nck1 but not of Nck2 or c-Cbl protein abundance ( Fig. 2a ). The quantitative analysis showed that Nck1 protein abundance was significantly lower in undifferentiated ( n =3, 17.0±3.2% s.e.m.) and synaptopodin-depleted differentiated podocytes ( n =3, 26.1±3.5 %) but not in control shRNA-infected differentiated podocytes (98.6±3.5 %) when compared with synaptopodin-replete differentiated podocytes ( P <0.001, analysis of variance (ANOVA); Fig. 2b ). In contrast, the Nck2 protein abundance was not altered by the presence or absence of synaptopodin (undifferentiated podocytes: n =3, 113.9±17.6%, synaptopodin shRNA-infected cells: n =3, 104.7±13.7, control shRNA-infected cells: n =3, 82.3±10.5%; Fig. 2b ). These results suggested that the depletion of synaptopodin causes a reduction in Nck1 protein abundance. Consistent with this hypothesis, transfection of undifferentiated podocytes with GFP-Synpo-long but not the GFP-sui control increased Nck1 protein abundance ( Fig. 2c ). In contrast, Nck2 protein abundance was unaffected ( Fig. 2c ). These data hinted at a coordinate functional relationship between synaptopodin and Nck1 (but not Nck2), which we set out to explore further. 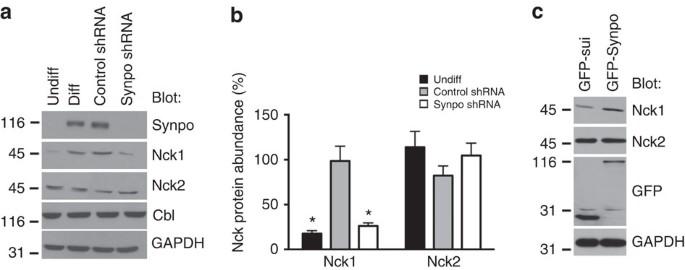Figure 2: Synaptopodin increases the protein abundance of Nck1 but not Nck2. (a) Synaptopodin is not expressed in undifferentiated (undiff) podocytes and is markedly downregulated in synaptopodin knockdown podocytes (synpo shRNA), when compared with differentiated (diff) and non-silencing shRNA control cells. Similarly, Nck1 protein levels are low in undifferentiated and synaptopodin knockdown podocytes. Nck2 levels are comparable under all conditions. GAPDH serves as a loading control. (b) Quantification of Nck1 and Nck2 protein abundance in the presence or absence of synaptopodin. Statistical analysis was performed by pairwise comparison of undifferentiated versus differentiated podocytes, or scrambled shRNA versus synaptopodin shRNA-infected cells using Student’st-test. Values are presented as % band intensity of differentiated podocytes ±s.e.m.,n=3, *P<0.05. (c) Transfection of undifferentiated podocytes with GFP-Synpo-long but not GFP-sui (negative control) increases Nck1 but not Nck2 protein abundance. GAPDH serves as loading control. Molecular weight markers are in kDa. Figure 2: Synaptopodin increases the protein abundance of Nck1 but not Nck2. ( a ) Synaptopodin is not expressed in undifferentiated (undiff) podocytes and is markedly downregulated in synaptopodin knockdown podocytes (synpo shRNA), when compared with differentiated (diff) and non-silencing shRNA control cells. Similarly, Nck1 protein levels are low in undifferentiated and synaptopodin knockdown podocytes. Nck2 levels are comparable under all conditions. GAPDH serves as a loading control. ( b ) Quantification of Nck1 and Nck2 protein abundance in the presence or absence of synaptopodin. Statistical analysis was performed by pairwise comparison of undifferentiated versus differentiated podocytes, or scrambled shRNA versus synaptopodin shRNA-infected cells using Student’s t -test. Values are presented as % band intensity of differentiated podocytes ±s.e.m., n =3, * P <0.05. ( c ) Transfection of undifferentiated podocytes with GFP-Synpo-long but not GFP-sui (negative control) increases Nck1 but not Nck2 protein abundance. GAPDH serves as loading control. Molecular weight markers are in kDa. Full size image Synaptopodin increases Nck1 protein abundance Synaptopodin can prevent the proteasomal degradation of RhoA by blocking the binding of Smurf1 to RhoA [13] . Nck can bind to c-Cbl [18] ; therefore, we reasoned that c-Cbl may target Nck1 for proteasomal degradation and that, similar to the inhibition of RhoA ubiquitination by Smurf1 (ref. 13 ), synaptopodin can prevent the ubiquitination of Nck1 by c-Cbl. Consistent with this hypothesis, treatment of synaptopodin knockdown podocytes with the proteasome inhibitor lactacystin induced the upregulation of Nck1 and cyclin D1 (serving as positive control for proteasome inhibition [13] ) steady-state protein levels ( Fig. 3a ), thereby showing that a pool of Nck1 is ubiquitinated and targeted to the proteasome. Quantitative analysis revealed that Nck1 protein abundance was significantly lower in synaptopodin-depleted cells ( n =3, 45.0±7.9% s.e.m.) compared with lactacystin-treated synaptopodin-depleted cells ( n =3, 100.7±16.3%; P <0.05, ANOVA; Fig. 3b ). Treatment of control shRNA-infected cells with lactacystin did not change Nck1 protein abundance ( n =3, 100.3±8.9%). Nck2 levels were not changed by lactacystin in control shRNA-infected cells ( n =3, 115.7±13.2%), synaptopodin shRNA-infected cells (106.2±24.1%) or untreated synaptopodin shRNA-infected cells ( n =3, 92.3±17.6%) ( Fig. 3b ). 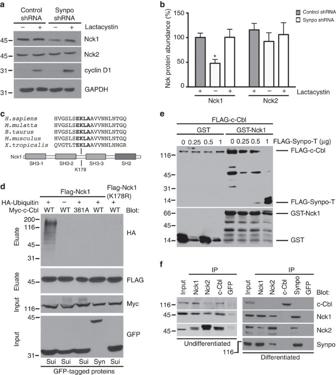Figure 3: c-Cbl-mediated ubiquitination of Nck1 is blocked by competitive binding of synaptopodin to Nck1. (a) Lactacystin increases Nck1 and cyclin D1 (positive control) steady-state protein levels in synaptopodin knockdown podocytes. Nck2 protein abundance remains unchanged. GAPDH serves as loading control. (b) Quantification of lactacystin induced changes in Nck1 and Nck2 abundance in synaptopodin-depleted podocytes. Values are presented as % of untreated control shRNA-expressing cells ±s.e.m.,n=3, ANOVA, *P<0.05. (c) Nck1 contains a lysine at position 178 that is conserved fromXenopusto human. (d) FLAG-Nck1 is ubiquitinated by wild-type (WT) but not by catalytically inactive (381A) c-Cbl in transfected HEK cells co-expressing GFP-sui, as revealed using anti-HA immunoblotting. GFP-Synpo-T (Syn) but not GFP-sui blocks the ubiquitination of Nck1. Nck1(K178R) is resistant to ubiquitination by c-Cbl. No ubiquitination is detected in the absence of HA-ubiquitin. (e) Immobilized GST-Nck1 directly binds to purified FLAG-c-Cbl. In the presence of increasing amounts of FLAG-Synpo-T, binding of Nck1 to c-Cbl is gradually lost, whereas increased binding of Synpo-T to Nck1 is detected. (f) Endogenous Nck1 and Nck2 co-precipitate with c-Cbl in undifferentiated (non-synaptopodin containing) podocytes. In differentiated (synaptopodin replete) podocytes, Nck1 (and Nck2) binds to synaptopodin at the expense of c-Cbl. No interaction is found between c-Cbl and synaptopodin. Molecular weight markers are in kDa. Figure 3: c-Cbl-mediated ubiquitination of Nck1 is blocked by competitive binding of synaptopodin to Nck1. ( a ) Lactacystin increases Nck1 and cyclin D1 (positive control) steady-state protein levels in synaptopodin knockdown podocytes. Nck2 protein abundance remains unchanged. GAPDH serves as loading control. ( b ) Quantification of lactacystin induced changes in Nck1 and Nck2 abundance in synaptopodin-depleted podocytes. Values are presented as % of untreated control shRNA-expressing cells ±s.e.m., n =3, ANOVA, * P <0.05. ( c ) Nck1 contains a lysine at position 178 that is conserved from Xenopus to human. ( d ) FLAG-Nck1 is ubiquitinated by wild-type (WT) but not by catalytically inactive (381A) c-Cbl in transfected HEK cells co-expressing GFP-sui, as revealed using anti-HA immunoblotting. GFP-Synpo-T (Syn) but not GFP-sui blocks the ubiquitination of Nck1. Nck1(K178R) is resistant to ubiquitination by c-Cbl. No ubiquitination is detected in the absence of HA-ubiquitin. ( e ) Immobilized GST-Nck1 directly binds to purified FLAG-c-Cbl. In the presence of increasing amounts of FLAG-Synpo-T, binding of Nck1 to c-Cbl is gradually lost, whereas increased binding of Synpo-T to Nck1 is detected. ( f ) Endogenous Nck1 and Nck2 co-precipitate with c-Cbl in undifferentiated (non-synaptopodin containing) podocytes. In differentiated (synaptopodin replete) podocytes, Nck1 (and Nck2) binds to synaptopodin at the expense of c-Cbl. No interaction is found between c-Cbl and synaptopodin. Molecular weight markers are in kDa. Full size image Synaptopodin blocks the Cbl-mediated ubiquitination of Nck1 We next searched for preferred in vivo ubiquitination sites [19] present in Nck1 but not Nck2 and identified lysine 178, which is evolutionarily conserved from Xenopus to human ( Fig. 3c ). Therefore, we reasoned that lysine 178 of Nck1 could serve as acceptor for ubiquitin transferred by c-Cbl. To directly test this hypothesis, we mutated lysine 178 of Nck1 to arginine and analysed Nck1 ubiquitination using immunoprecipitation with anti-FLAG antibody in HEK293 co-transfected with FLAG-Nck1, FLAG-Nck1(K178R), Myc-c-Cbl (WT or catalytically inactive C381A [20] ) and HA-ubiquitin in the presence of GFP-Synpo-T or GFP-sui (negative control), respectively ( Fig. 3d ). No ubiquitination was found in cells lacking HA-ubiquitin or in cells expressing catalytically inactive c-Cbl (C381A). In cells expressing the GFP-sui control, FLAG-Nck1 was strongly ubiquitinated by c-Cbl ( Fig. 3d ). In contrast, co-expression of GFP-Synpo-T abrogated the ubiquitination of Nck1. Similarly, Nck1(K178R) was also protected from c-Cbl-mediated ubiquitination ( Fig. 3d ). We also probed the western blot membrane with anti-Nck1 and found that the high molecular weights were in fact Nck1 ( Supplementary Fig. S1 ). Taken together, these results show that lysine 178 in Nck1 is the acceptor site for ubiquitin transferred by c-Cbl, and that the ubiquitination of Nck1 by c-Cbl is blocked in the presence of synaptopodin. c-Cbl and synaptopodin compete for Nck1 binding To directly test whether synaptopodin prevents the ubiquitination of Nck1 by competing with c-Cbl for Nck1 binding, we conducted in vitro reconstitution studies according to our previously published protocols [13] , [21] . We immobilized 1 μg purified GST-Nck1 on glutathione (GSH) beads and incubated it with 1 μg of purified FLAG-c-Cbl and increasing amounts (0, 0.25, 0.5 or 1 μg) of FLAG-Synpo-T ( Fig. 3e ). In the absence of Synpo-T, c-Cbl strongly bound to GST-Nck1 but only weakly to the GST control. In contrast, the binding of Synpo-T to GST-Nck1 decreased the binding of FLAG-c-Cbl to GST-Nck1 in a concentration-dependent manner ( Fig. 3e ). In the presence of 1 μg of Synpo-T, minimal, if any, binding of c-Cbl to Nck1 could be detected ( Fig. 3e ). To confirm the physiologic relevance of synaptopodin-mediated inhibition of c-Cbl binding to Nck1, we conducted endogenous Co-IP studies with extracts from undifferentiated and differentiated cultured podocytes ( Fig. 3f ). In undifferentiated podocytes lacking synaptopodin, c-Cbl interacted with Nck1 and Nck2 ( Fig. 3f , left panel). In contrast, in synaptopodin-expressing differentiated podocytes, synaptopodin interacted with Nck1 and Nck2, at the expense of their interaction with c-Cbl ( Fig. 3f , right panel). Of note, c-Cbl did not interact with synaptopodin ( Fig. 3f , right panel). Altogether, these data unveil Nck1 as a target of c-Cbl-mediated ubiquitination and ensuing proteasomal degradation. c-Cbl depletion restores Nck1 protein abundance Nck and synaptopodin are both involved in the regulation of actin dynamics [7] . Gene silencing of synaptopodin causes a loss of RhoA signalling and stress fibres [13] , as well as a reduction in Nck1 protein abundance ( Fig. 2a ). The loss of stress fibres in synaptopodin-deficient podocytes can be rescued by overexpression of Smurf1-resistant RhoA(K6,7R) [13] . To test the effect of c-Cbl-resistant Nck1(K178R) on actin dynamics, we infected synaptopodin knockdown podocytes with GFP-Nck1, GFP-Nck1(K178R), GFP-Nck2 or GFP alone. We validated the expression of all four GFP-tagged proteins and the efficiency of synaptopodin depletion using western blot ( Fig. 4a ). Of note, the shRNA-mediated loss of synaptopodin was not affected by the ectopic expression of the various GFP constructs ( Fig. 4a ). In a complementary approach, we infected synaptopodin-depleted podocytes with c-Cbl shRNA or a scrambled control shRNA and analysed Nck1 protein abundance using western blot ( Fig. 4b ). We found that the synaptopodin depletion-mediated reduction in Nck1 protein abundance was rescued by gene silencing of c-Cbl ( Fig. 4b ). Quantitative analysis revealed significantly higher Nck1 protein abundance in synaptopodin/c-Cbl co-depleted podocytes ( n =3, 77.4±6.4% s.e.m.) compared with synaptopodin-depleted podocytes ( n =3, 19.3±3.0%), P <0.01, t -test ( Fig. 4c ). In contrast, Nck2 protein abundance was comparable in synaptopodin-depleted ( n =3, 96.7±11. 2 %) and synaptopodin/c-Cbl-co-depleted podocytes ( n =3, 99.7±12.6%; Fig. 4c ). These data confirm that c-Cbl is required for the decreased Nck1 protein abundance in synaptopodin-depleted podocytes. 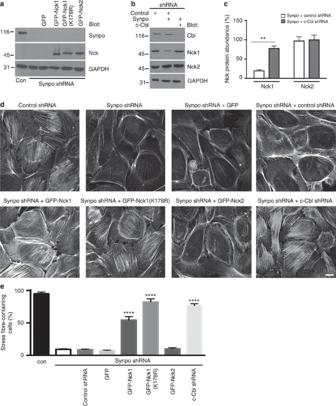Figure 4: Gene silencing of c-Cbl or overexpression of Nck1 rescues stress fibre formation in synaptopodin-depleted podocytes. (a) Western blot analysis confirms synaptopodin depletion in synaptopodin knockdown (synpo shRNA) podocytes compared with cells expressing a non-silencing control shRNA (con). Western blot for Nck shows comparable expression levels of GFP-Nck1, GFP-Nck1(K178R) and GFP-Nck2 in synaptopodin knockdown cells. (b) Western blots analysis confirms the rescue of Nck1 protein abundance in synaptopodin knockdown podocytes by gene silencing of c-Cbl shRNA. Nck2 levels are comparable under all conditions. GAPDH serves as a loading control. (c) Quantification of Nck1 and Nck2 protein abundance in c-Cbl-depleted synaptopodin shRNA cells. Values are presented as % of control shRNA band intensity±s.e.m.,n=3, ANOVA, **P<0.01. (d) Phalloidin labelling shows the loss of stress fibres in synaptopodin knockdown (synpo shRNA) but not in control shRNA-infected cells. GFP-Nck1 and GFP-Nck1(K178R) but not GFP-Nck2 or GFP alone restore stress fibres. Gene silencing of c-Cbl but not a control shRNA also restore stress fibres in synaptopodin-depleted podocytes. Scale bar 20 μM (e) Quantitative analysis shows a partial rescue of stress fibre formation by GFP-Nck1 and a complete rescue by GFP-Nck1(K178R) or c-Cbl shRNA. Values are presented as % stress fibre-containing cells ±s.e.m.,n=3, ANOVA, ****P<0.0001. Molecular weight markers are in kDa. Figure 4: Gene silencing of c-Cbl or overexpression of Nck1 rescues stress fibre formation in synaptopodin-depleted podocytes. ( a ) Western blot analysis confirms synaptopodin depletion in synaptopodin knockdown (synpo shRNA) podocytes compared with cells expressing a non-silencing control shRNA (con). Western blot for Nck shows comparable expression levels of GFP-Nck1, GFP-Nck1(K178R) and GFP-Nck2 in synaptopodin knockdown cells. ( b ) Western blots analysis confirms the rescue of Nck1 protein abundance in synaptopodin knockdown podocytes by gene silencing of c-Cbl shRNA. Nck2 levels are comparable under all conditions. GAPDH serves as a loading control. ( c ) Quantification of Nck1 and Nck2 protein abundance in c-Cbl-depleted synaptopodin shRNA cells. Values are presented as % of control shRNA band intensity±s.e.m., n =3, ANOVA, ** P <0.01. ( d ) Phalloidin labelling shows the loss of stress fibres in synaptopodin knockdown (synpo shRNA) but not in control shRNA-infected cells. GFP-Nck1 and GFP-Nck1(K178R) but not GFP-Nck2 or GFP alone restore stress fibres. Gene silencing of c-Cbl but not a control shRNA also restore stress fibres in synaptopodin-depleted podocytes. Scale bar 20 μM ( e ) Quantitative analysis shows a partial rescue of stress fibre formation by GFP-Nck1 and a complete rescue by GFP-Nck1(K178R) or c-Cbl shRNA. Values are presented as % stress fibre-containing cells ±s.e.m., n =3, ANOVA, **** P <0.0001. Molecular weight markers are in kDa. Full size image c-Cbl-resistant Nck1(K178R) restore stress fibres We then visualized the actin cytoskeleton by phalloidin labelling ( Fig. 4d ). Similar to synaptopodin-depleted cells, few cells infected with GFP-Nck2 or the GFP control contained stress fibres. In contrast, GFP-Nck1 and, even more robustly, c-Cbl-resistant GFP-Nck1(K178R) induced stress fibres in synaptopodin-depleted cells ( Fig. 4d ). We also observed the rescue of stress fibres in synaptopodin-depleted podocytes co-infected with c-Cbl shRNA but not a non-silencing control shRNA ( Fig. 4d , right). Quantitative analysis ( Fig. 4e ) showed a partial rescue of stress fibres with GFP-Nck1 and a complete rescue with GFP-Nck1(K178R) or c-Cbl shRNA (control shRNA: n =3, 95.0±2.5% s.e.m. stress fibre-containing cells; synpo shRNA: n =3, 9.3±0.9%; synpo shRNA+control shRNA: n =3, 8.8±0.9%; synpo shRNA+GFP: n =3, 7.4.±0.7%; synpo shRNA + GFP-Nck1: n =3, 54.5±5.3%; synpo shRNA+GFP-Nck1(K178R): n =3, 82.5±4.6%; synpo shRNA+GFP-Nck2: n =3, 10.0.±1.8%; synpo shRNA±c-Cbl shRNA: n =3, 76.7±2.8%; P <0.0001, ANOVA). Taken together, c-Cbl-mediated ubiquitination of Nck1 causes the loss of stress fibres in podocytes, an effect that can be blocked by synaptopodin. Nck1 signals through Rho kinase and formin Nck can interact with N-WASP to promote Arp2/3-mediated actin nucleation [3] , [4] . In endothelial cells, Nck-mediated activation of Arp2/3 contributes to stress fibre formation [22] . Nck can also regulate RhoA signalling, and mouse embryonic fibroblast lacking Nck show impaired Rho GTPase activation downstream of platelet-derived growth factor β receptor [23] . To test whether Nck1-induced stress fibre formation in synaptopodin-depleted podocytes resulted from the activation of RhoA (and its downstream effectors including Rho kinase and formins) or from the activation of N-WASP/Arp2/3 signalling, we examined the effects of the Arp2/3 blocker CK666 (ref. 24 ), the formin inhibitor SMIFH2 (ref. 25 ) and the Rho kinase inhibitor Y27632 (ref. 26 ) on stress fibres in podocytes expressing a non-silencing control shRNA+GFP versus synpo shRNA+GFP-Nck1(K178R). Synaptopodin-depleted podocytes rescued by expression of Smurf1-resistant GFP-RhoA(K6,7R) [13] served as positive control ( Fig. 5a ). Podocytes infected with the control shRNA + GFP showed well-developed stress fibres, which were blocked by SMIFH2 and Y27632, but not by CK666 ( Fig. 5a , upper panel). Similarly, synaptopodin-depleted podocytes infected with GFP-Nck1(K178R) ( Fig. 5a , middle panel) or Smurf1-resistant GFP-RhoA(K6,7R) ( Fig. 5a , lower panel) showed well-developed stress fibres, which were suppressed by SMIFH2 or Y27632, but not by CK666. To confirm that the CK666 compound used in these studies was active and capable of disrupting Arp2/3 complexes [24] , we visualized the effect of CK666 on ARP3 expression using confocal microscopy. In keeping with published studies [27] , CK666 caused the loss of ARP3 expression but had no effect on stress fibre integrity ( Fig. 5b ), thereby confirming that CK666 was active. The quantitative analysis ( Fig. 5c ) confirmed the loss of stress fibres in cells treated with SMIFH2 or Y27632 but not CK666 (control shRNA+GFP: n =3, 88.4±1.7% s.e.m. stress fibre-containing cells; synpo shRNA+GFP-Nck1(K178R): n =3, 87.4±3.2%; synpo shRNA+RhoA(K6,7R): 85.6±3.4%; control shRNA+GFP+CK666: n =3, 82.2±2.6%; synpo shRNA+GFP-Nck1(K178R)+CK666: n =3, 85.8±2.7%; synpo shRNA+RhoA(K6,7R)+CK666: n =3, 84.7±7.3%; control shRNA+GFP+SMIFH2: n =3, 3.1±0.9%; synpo shRNA+GFP-Nck1(K178R)+SMIFH2: n =3, 3.7±0.2%; synpo shRNA+RhoA(K6,7R)+SMIFH2: n =3, 6.9±0.6%; control shRNA+GFP+Y27632: n =3, 5.6±1.9%; synpo shRNA+GFP-Nck1(K178R)+Y27632: n =3, 2.1±1.1 %; synpo shRNA+RhoA(K6,7R)+Y27632: n =3, 1.3±1.3%; P <0.0001, ANOVA). 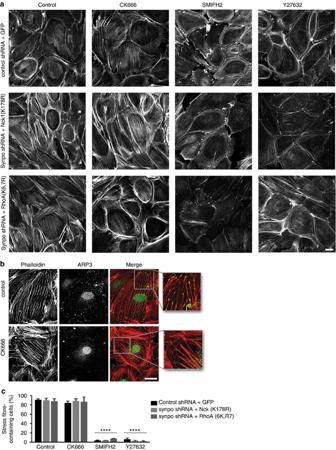Figure 5: Nck1 promotes stress fibre formation via Rho kinase and formin signalling. (a) Phalloidin labelling shows well-developed stress fibres in podocytes infected with a non-silencing control shRNA and GFP, and in synaptopodin knockdown (synpo shRNA) podocytes infected with GFP-Nck1(K178R) or GFP-RhoA(K6,7R). The Arp2/3 inhibitor CK666 does not disrupt stress fibres. In contrast, the formin inhibitor SMIFH2 or the Rho kinase inhibitor Y27632 cause a loss of stress fibres in control shRNA-infected cells and synaptopodin knockdown podocytes infected with GFP-Nck1(K178R) or GFP-RhoA(K6,7R). Scale bar 20 μM (b) Double labelling for phalloidin and ARP3 confirms the loss of ARP3 in CK666-treated podocytes but not in dimethylsulphoxide-treated control cells without affecting stress fibre integrity. Scale bar 20 μM (c) Quantitative analysis showing a significant loss of stress fibres after SMIFH2 (formin inhibitor) or Y-27632 (Rho kinase inhibitor) treatment. Values are presented as % stress fibre-containing cells ±s.e.m.,n=3, ANOVA, ****P<0.0001. Figure 5: Nck1 promotes stress fibre formation via Rho kinase and formin signalling. ( a ) Phalloidin labelling shows well-developed stress fibres in podocytes infected with a non-silencing control shRNA and GFP, and in synaptopodin knockdown (synpo shRNA) podocytes infected with GFP-Nck1(K178R) or GFP-RhoA(K6,7R). The Arp2/3 inhibitor CK666 does not disrupt stress fibres. In contrast, the formin inhibitor SMIFH2 or the Rho kinase inhibitor Y27632 cause a loss of stress fibres in control shRNA-infected cells and synaptopodin knockdown podocytes infected with GFP-Nck1(K178R) or GFP-RhoA(K6,7R). Scale bar 20 μM ( b ) Double labelling for phalloidin and ARP3 confirms the loss of ARP3 in CK666-treated podocytes but not in dimethylsulphoxide-treated control cells without affecting stress fibre integrity. Scale bar 20 μM ( c ) Quantitative analysis showing a significant loss of stress fibres after SMIFH2 (formin inhibitor) or Y-27632 (Rho kinase inhibitor) treatment. Values are presented as % stress fibre-containing cells ±s.e.m., n =3, ANOVA, **** P <0.0001. Full size image Nck1 increases RhoA activation and cofilin phosphorylation Our data presented so far suggested that Nck1 restores stress fibres in synaptopodin-depleted podocytes through the activation of Rho kinase and formin-mediated signalling downstream of RhoA activation. To test this directly, we performed RhoA activity assays. Consistent with our hypothesis, GFP-Nck1 and more strikingly c-Cbl-resistant GFP-Nck1(K178R) but not GFP-Nck2, increased RhoA activation as well as downstream cofilin phosphorylation [28] in synaptopodin-depleted podocytes ( Fig. 6a ). The quantitative analysis revealed significantly increased RhoA activity in synaptopodin-depleted podocytes expressing c-Cbl-resistant Nck1(K178R) ( n =3, 184.3± 50.2% s.e.m.) but not in synaptopodin-depleted podocytes expressing GFP ( n =3, 27.6±2.1 5%), GFP-Nck1: ( n =3, 80.4±30.8%) or GFP-Nck2 ( n =3, 20.8±1.9%) when compared with control shRNA-expressing or synaptopodin-depleted cells ( n =3, 13.3±3.3%), P <0.001, ANOVA ( Fig. 6b ). Phosphorylated cofilin protein abundance was also significantly increased in synaptopodin-depleted podocytes expressing c-Cbl-resistant Nck1(K178R) ( n =3, 191± 24.8% s.e.m.) when compared with control shRNA expressing or synaptopodin-depleted cells ( n =3, 51.3±1.8 %), or synaptopodin-depleted cells expressing GFP ( n =3, 39.3±6.7%) synpo shRNA GFP-Nck1 ( n =3, 99.7±12.7%) or GFP-Nck2 ( n =3, 38.0±3.2%); P <0.0001, ANOVA ( Fig. 6c ). These results confirm that the induction of stress fibres by c-Cbl-resistant Nck1 is because of downstream activation of RhoA. 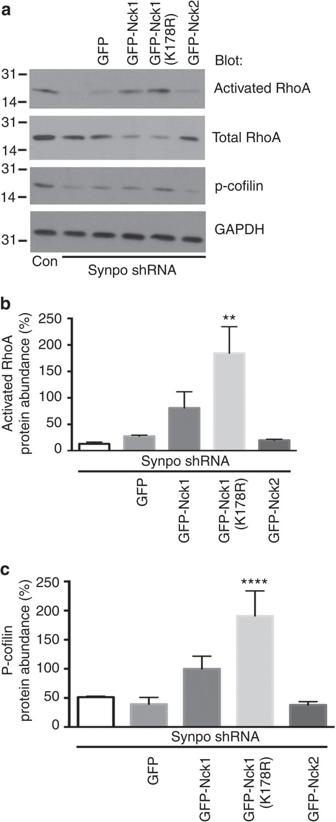Figure 6: Nck1 increases RhoA activation and cofilin phosphorylation. (a) GFP-Nck1 and more strongly c-Cbl-resistant GFP-Nck1(K178R) but GFP-Nck2 or GFP alone increase the abundance of GTP-bound active RhoA and the downstream target phospho-cofilin. GAPDH serves as loading control. Molecular weight markers are in kDa. (b) Quantitative analysis of RhoA activation in synaptopodin-depleted cells overexpressing c-Cbl-resistant GFP-Nck1 (K178R), **P<0.01. Data are presented as % ±s.e.m. of control shRNA-expressing cells,n=3. (c) Quantitative analysis of p-cofilin abundance in synaptopodin-depleted cells overexpressing GFP-Nck1 (K178R). Data are presented as % ±s.e.m. of control shRNA-expressing cells,n=3, ANOVA, ****P<0.0001. Figure 6: Nck1 increases RhoA activation and cofilin phosphorylation. ( a ) GFP-Nck1 and more strongly c-Cbl-resistant GFP-Nck1(K178R) but GFP-Nck2 or GFP alone increase the abundance of GTP-bound active RhoA and the downstream target phospho-cofilin. GAPDH serves as loading control. Molecular weight markers are in kDa. ( b ) Quantitative analysis of RhoA activation in synaptopodin-depleted cells overexpressing c-Cbl-resistant GFP-Nck1 (K178R), ** P <0.01. Data are presented as % ±s.e.m. of control shRNA-expressing cells, n =3. ( c ) Quantitative analysis of p-cofilin abundance in synaptopodin-depleted cells overexpressing GFP-Nck1 (K178R). Data are presented as % ±s.e.m. of control shRNA-expressing cells, n =3, ANOVA, **** P <0.0001. Full size image SH3 domain 2 of Nck1 is required for stress fibre formation To start exploring why Nck1, but not the highly homologous Nck2, is capable of inducing stress fibres, we conducted domain-swapping experiments with chimeric proteins using Nck2 constructs containing SH3 domains 1, 2 or 3 or the SH2 domain of Nck1 ( Fig. 7a ). Of note, the Nck1-specific ubiquitination site (K178) is not present in any of the chimeric constructs. We validated the expression of all four GFP-tagged chimeric proteins as well as GFP-Nck1(K178R) and GFP-Nck2 using western blot ( Fig. 7b ). Similar to Nck1(K178R), Nck2/Nck1 SH3-2 containing the second SH3 domain of Nck1, but none of the other chimeric constructs, induced stress fibres in synaptopodin-depleted cells ( Fig. 7c ). Quantitative analysis showed a significant rescue of stress fibres by Nck2/Nck1 SH3-2 or c-Cbl-resistant Nck1 (K178R); GFP-Nck1(K178R): n =3, 82.9±2.2% s.e.m. ; GFP-Nck2: n =3, 14.9±0.9%; GFP-Nck2/Nck1 SH3-1: 15.3±1.3%; GFP-Nck2/Nck1 SH3-2: n =3, 62.4±2.0%; Nck2/Nck1 SH3-3: n =3, 14.4±0.6%; Nck2/Nck1 SH2: n =3, 14.1±0.8%, P <0.0001, ANOVA ( Fig. 7d ). These data reveal that the second SH3 domain mediates the effects of Nck1 on stress fibre assembly. Importantly, they also offer a molecular explanation why Nck2 cannot induce stress fibres, despite its overall homology to Nck1. 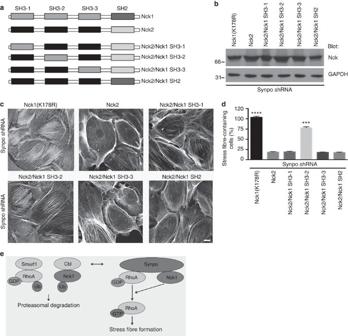Figure 7: SH3 domain 2 in Nck1 is essential for stress fibre formation. (a) Schematic showing the domain structure of Nck1, Nck2 and four Nck2 constructs containing Nck1 domains. (b) Western blot for Nck shows comparable expression levels for GFP-Nck1(K178R), GFP-Nck2, GFP-Nck2/Nck1 SH3-1, GFP-Nck2/Nck1 SH2, GFP-Nck2/Nck1 SH3 and GFP-Nck2/Nck1 SH2 in synaptopodin knockdown cells. Molecular weight markers are in kDa. (c) Phalloidin labelling shows the induction of stress fibres in synaptopodin-depleted (synpo shRNA) cells expressing c-Cbl-resistant Nck1(K178R) or Nck2/Nck1 SH3-2. Scale bar 20 μM. (d) Quantitative analysis showing a significant increase in stress fibres containing synaptopodin-depleted cells expressing c-Cbl-resistant Nck1(K178R) or Nck2/Nck1 SH3-2. Values are presented as % stress fibre-containing cells ±s.e.m.,n=3, ANOVA ***P<0.001, ****P<0.0001. (e) A model for the co-regulation of RhoA signalling by Nck and synaptopodin. (Left) In the absence of synaptopodin, RhoA and Nck1 are targeted for proteasomal degradation by Smurf1-or c-Cbl, respectively. (Right) Synaptopodin (Synpo) prevents the targeting of RhoA and Nck1 for proteasomal degradation by blocking the binding of Smurf1 to RhoA and the binding of c-Cbl to Nck1, thereby increasing RhoA activation and stress fibre formation. Ub, ubiquitin. Figure 7: SH3 domain 2 in Nck1 is essential for stress fibre formation. ( a ) Schematic showing the domain structure of Nck1, Nck2 and four Nck2 constructs containing Nck1 domains. ( b ) Western blot for Nck shows comparable expression levels for GFP-Nck1(K178R), GFP-Nck2, GFP-Nck2/Nck1 SH3-1, GFP-Nck2/Nck1 SH2, GFP-Nck2/Nck1 SH3 and GFP-Nck2/Nck1 SH2 in synaptopodin knockdown cells. Molecular weight markers are in kDa. ( c ) Phalloidin labelling shows the induction of stress fibres in synaptopodin-depleted (synpo shRNA) cells expressing c-Cbl-resistant Nck1(K178R) or Nck2/Nck1 SH3-2. Scale bar 20 μM. ( d ) Quantitative analysis showing a significant increase in stress fibres containing synaptopodin-depleted cells expressing c-Cbl-resistant Nck1(K178R) or Nck2/Nck1 SH3-2. Values are presented as % stress fibre-containing cells ±s.e.m., n =3, ANOVA *** P <0.001, **** P <0.0001. ( e ) A model for the co-regulation of RhoA signalling by Nck and synaptopodin. (Left) In the absence of synaptopodin, RhoA and Nck1 are targeted for proteasomal degradation by Smurf1-or c-Cbl, respectively. (Right) Synaptopodin (Synpo) prevents the targeting of RhoA and Nck1 for proteasomal degradation by blocking the binding of Smurf1 to RhoA and the binding of c-Cbl to Nck1, thereby increasing RhoA activation and stress fibre formation. Ub, ubiquitin. Full size image The studies described here have allowed us to explore several important questions. c-Cbl was the first identified binding partner of the SH3 domain of Nck [29] . Since then, Nck has been described in several systems as an adapter molecule, binding to autophosphorylated receptor tyrosine kinases (RTKs) such as Abl at their phosphotyrosine residues to recruit Cbl via its SH3 domains [30] , [31] . At the cell membrane, RTKs are ubiquitinated by c-Cbl, resulting in their internalization (upon monoubiquitination) or proteasomal degradation (after polyubiquitination) [32] . Here we make the unanticipated observation that Nck1 but not Nck2 is a substrate of c-Cbl-mediated ubiquitination and subsequent proteasomal degradation. We have identified lysine 178 as the ubiquitin acceptor site, which is conserved from Xenopus to human, underscoring the physiologic relevance of Nck1 ubiquitination. It is intriguing to speculate that proteasomal regulation enables Nck1 (and not Nck2) to mediate spatially and temporally restricted changes in RhoA-induced actin dynamics. This notion is supported by the observation that the Nck1 stabilizer synaptopodin has both a short half-life [15] , which enables it to mediate dynamic cytoskeletal changes [15] , and is itself regulated by TRPC5/Ca 2+ and calcineurin-dependent degradation [33] , [34] . Previous studies revealed a role for c-Cbl as a negative regulator of Arp2/3-mediated actin polymerization through the ubiquitination of phosphorylated mDab1 (ref. 35 ) or WAVE2 (ref. 36 ), respectively. Our data extend these findings, elucidating c-Cbl as a negative regulator of Nck1-induced, formin-mediated actin polymerization. By uncovering the synaptopodin-mediated protection of Nck1 from c-Cbl-mediated ubiquitination, we have revealed a role for Nck1 in stress fibre formation by an Arp2/3-independent but Rho kinase- and formin-dependent mechanism. Nck1 and Nck2 are known to have overlapping but also non-redundant functions [1] —for example, PAK preferably interacts with Nck2 to downregulate synaptic transmission [37] . Moreover, epidermal growth factor receptor and platelet-derived growth factor receptor preferentially interact with Nck2 (ref. 38 ). This points to differences in specific binding affinities between Nck1 and Nck2, despite overall sequence homology between these proteins [38] . We now provide evidence for a non-redundant function of Nck1 by showing that the second SH3 domain of Nck1 but not of Nck2 is involved in the regulation of stress fibre formation. These results are in keeping with previous findings that Nck1 can rescue actin filament formation in Nck1/Nck2 double null mouse embryonic fibroblasts [39] . Clearly, future studies are warranted to identify putative guanine exchange factors, GTPase-activating proteins or guanine nucleotide-dissociation inhibitors [28] that can bind to the second SH3 domain of Nck1 and mediate the observed activation of RhoA and stress fibre formation. In conclusion, our results reveal Nck1 but not Nck2 as a target of c-Cbl-mediated ubiquitination and proteasomal degradation. Furthermore, they identify synaptopodin as a putative general inhibitor of E3 ligases, including Smurf1 (ref. 13 ) and c-Cbl ( Fig. 7e ). Accordingly, Nck1 cooperates with synaptopodin in the regulation of RhoA. Taken together, our findings extend our understanding of the spatial and temporal regulation of the actin cytoskeleton. In addition to guanine nucleotide exchange factors, GTPase-activating proteins [13] , RhoGDI [40] , or ubiquitination of RhoA [13] , [15] , [41] , c-Cbl-mediated ubiquitination of Nck1 is now revealed as an additional, critical component of the ever expanding signalling machinery that regulates Rho proteins and actin dynamics. Plasmid constructs HA-tagged human Nck1 and Nck2 cDNAs in the PRK5 vector were kindly provided by Wei Li and cloned into pEGFP-N1 (CLONTECH), pFLAG-CMV-5a,b,c (Sigma-Aldrich) or a modified Glutathione S-transferase fusion vector (pGEX). HA-tagged c-Cbl cDNA in pCEFL was provided by Stanley Lipkowitz and subcloned into pFLAG-CMV-5a or pcDNA 3.1/Myc-His A vector, HA-ubiquitin was provided by Keiji Tanaka. FLAG-synaptopodin constructs (Synpo-long, Synpo-short and Synpo-T) have been described previously [12] . The QuikChange Multi Site-Directed Mutagenesis Kit (STRATAGENE) was used according to the manufacturer’s protocol to generate the K178R amino-acid substitution in Nck1 using GFP-Nck1 or FLAG-Nck1 as template. The same procedure was used to generate the catalytically inactive c-Cbl(C381A) [20] mutant using Myc-c-Cbl as template. All constructs were verified by DNA sequencing. The sequences of primers used for site-directed mutagenesis experiments are shown in Supplementary Table S1 . Domain swapping To exchange SH3 or SH2 domains between Nck1 and Nck2, a three-step approach was employed. The QuikChange Lightning Site-Directed Mutagenesis Kit (Agilent Technologies) was used according to the manufacture’s protocols to introduce deletions and insertions. First, the targeted domain was deleted using VVPW-EGFP-Nck2 as template. Then the corresponding Nck1 domain was generated with PCR using VVPW-EGFP-Nck1 as template. Finally, the Nck1 domain containing PCR product was introduced into the Nck2 domain-deleted constructs. The sequences of primers used for deletion and insertion experiments are shown in Supplementary Table S1 . All constructs were verified by DNA sequencing. The amino acids that were exchanged between Nck2 and Nck1 are shown in Supplementary Table S2 . Using this approach, the following chimeric constructs were generated ( Fig. 7a ): Nck2/Nck1 SH3-1, Nck2/Nck1 SH3-2, Nck2/Nck1 SH3-3 and Nck2/Nck1 SH2. Lentivirus production and infection of differentiated synaptopodin-depleted podocytes was performed as described below. Cell culture and transient transfection Conditionally immortalized murine podocytes [17] were propagated at 33 °C in RPMI 1640 containing 10 % fetal bovine serum (Invitrogen), 100 U ml −1 penicillin (Invitrogen), 100 μg ml −1 streptomycin (Invitrogen) and 10 U ml −1 recombinant mouse γ-interferon (Cell Sciences) to induce synthesis of the immortalizing T-antigen. Subcultivation was performed with trypsin at 37 °C after cells had reached confluence. Cells were passaged after 1:10 dilution. To initiate differentiation, podocytes were thermoshifted to 37 °C and were maintained in a medium without γ-interferon for 10–14 days. Transient transfection of undifferentiated podocytes or HEK293 cells using FuGene 6 Reagent (Roche) was performed according to the manufacturer’s instructions at a 1:3 DNA:Fugene ratio. Transfection mixture was added to cells and protein collection was performed 48 h post transfection. For proteasome inhibition, podocytes were treated for 8 h with 2.5 μM lactacystin (BD) [13] . The Rho kinase inhibitor Y-27632 (ref. 26 ) (5 μM), the formin inhibitor SMIFH2 (ref. 25 ) (10 μM) or the ARP2/3 inhibitor CK-666 (ref. 24 ) (100 μM) were applied for 90 min before cells were fixed and processed for phalloidin labelling of F-actin. Lentiviral gene silencing and overexpression Lentivirus-mediated gene silencing of synaptopodin or c-Cbl was performed according to recently described protocols [33] with some modifications. Synaptopodin shRNA hairpins were designed using the RNAi consortiums hairpin design protocol of the Harvard–Massachusetts Institute of Technology Broad Institute ( http://www.broadinstitute.org/rnai/public ) and cloned into pLKO.1 vector. The c-Cbl hairpins in pLKO.1 were purchased from Sigma-Aldrich. For lentivirus production, HEK293T cells were co-transfected with plko.1 encoding the shRNA, the packaging plasmid pMDG.2 ΔR8.91 and the envelope plasmid pCMV VSV-G at a ratio of 10:10:1 using Fugene (Promega). The medium was replaced at 18 h following transfection and harvest medium was collected after 48 h 33 . Five different synaptopodin and five different c-Cbl shRNAs were screened using western blotting for knockdown efficiency. The sequences of the shRNAs that were chosen for the knockdown experiments are shown in Supplementary Table S3 . The two shRNAs for synaptopodin (Synpo1 and Synpo2) were pooled and used in combination to target all three synaptopodin isoforms [12] . The c-Cbl shRNA worked efficiently alone. A non-silencing scrambled shRNA served as a control [33] . For lentivurs-mediated protein overexpression studies, HEK293T cells were transfected with the VVPW encoding the cDNA together with pMDG.2 ΔR8.91 and pCMV VSV-G at a ratio of 3:2:1 using Fugene transfection reagent (Promega). The collection of lentivirus-containing medium was performed in the same way as described above for the plko.1 protocol. Podocytes were infected on day 9 of differentiation with 4 μg ml −1 polybrene-containing virus media. When two infections were performed, they were preformed on 2 consecutive days, the first infection was performed on day 9 followed by the second infection on day 10 of differentiation. Podocytes were collected or stained at 96 h after the first infection. Western Blot and immunoprecipitation SDS–PAGE and western blotting were performed after collecting podocytes by scraping in CHAPS buffer (20 mM Tris pH 7.5, 500 mM NaCl, 0,5% CHAPS) or by scraping HEK293 cells in Triton buffer (50 mM Tris pH 7.5, 150 mM NaCl, 1% Triton), supplemented with protease inhibitors (Roche) and phosphatase inhibitors (Sigma), followed by lysis on ice for 30 min. Lysates were clarified using centrifugation at 18,000 × g for 15 min at 4 °C, and protein content was measured using a commercial BCA assay (Pierce). Equal amounts of protein were resolved in 8–10% bis-tris gels and electrotransferred to polyvinylidene diflouride membranes. For heterologous co-immunoprecipitation of fusion proteins [13] , [14] , [15] , HEK293 cells were co-transfected using Fugene transfection regent (Promega) and collected at 48 h after transfection. Endogenous co-immunoprecipitations were performed using cell lysates from isolated mouse glomeruli or cultured podocytes. Lysates were pre-cleared using 2 μl mouse or rabbit IgG-AC beads (Santa Cruz) for 1 h at 4 °C followed using centrifugation at 5,200 × g for 5 min at 4 °C. The supernatants were incubated with 40 μl agarose beads coated with anti-FLAG-M2 antibody (Sigma-Aldrich) at 4 °C overnight. Beads were collected using centrifugation for 1 min at 1,000 × g and washed five times using 1 ml IP buffer for 1 min on a rotor. Bound proteins were eluted by boiling in 50 μl Laemmli sample buffer at 95 °C for 5 min. In the ubiquitination experiments, Protein G-coupled magnetic beads (Invitrogen) were used for the immunoprecipitation of Flag-Nck1. Protein lysates were pre-incubated with anti-FLAG antibody (Sigma) for 4 h at 4 °C, followed by 1 h at 4 °C incubation with Protein G-coupled magnetic beads according to the manufacturer’s instructions. For western blotting, the following primary antibodies were used: anti-Nck (BD Biosciences, no. 610099), anti-Nck1 (Cell Signalling, no. 2319) and anti-Nck2 (Upstate, no. 07-100) were used at 1:1,000, anti-synaptopodin NT [11] at 1:5,000, anti-Cbl at 1:500 (Santa Cruz, no. B2607) anti-FLAG at 1:10,000 (Sigma, no. F3165), anti-HA (Cell Signalling, no. 3724) at 1:1,000, anti-c-Myc (Cell Signalling, no. 2278) at 1:1,000 and anti-GAPDH (EMD Millipore, no. CB1001) at 1:5,000. Secondary antibodies were horseradish peroxidase-conjugated conformation-specific mouse anti-rabbit (Cell Signalling, no. 5127), goat anti-mouse and goat anti-rabbit (Promega, no. W402B and no. W401B), which were used at 1:5,000, 1:10,000 and 20,000, respectively. Protein abundance was quantified by analysing the intensity of western blot bands using the Image J software. Protein abundance was then normalized against GAPDH. The data were obtained from three independent experiments. Uncropped scans of the most important western blots are shown in Supplementary Figs S2–S5 . RhoA activation assay Activated RhoA was measured with a commercial Rho activation assay kit (Upstate) using a GST-tagged fusion protein corresponding to residues 7–89 of mouse Rhotekin Rho-binding domain according to the manufacturer’s instructions. After the pull down, the eluted active RhoA was detected using immunoblotting as described above using a rabbit monoclonal RhoA (Cell Signalling no. 2117) antibody at 1:1,000. Total RhoA and GADPH were measured in the cell lysates used for the pull-down studies and served as loading controls. RhoA activity was calculated as active RhoA/total RhoA obtained from the quantification of three independent experiments. GST-binding assay The competitive binding of synaptopodin and c-Cbl to Nck1 was analysed in GST pull-down studies with purified recombinant proteins [13] , [14] , [15] . GST-tagged Nck proteins were expressed in bacteria and cultivated in LB medium to an OD600=0.8. To purify GST-Nck, 1 mM isopropyl-β-D-thiogalactopyranoside was added and bacteria were pelleted at 3,000 g for 10 min at 4 °C and resuspended in lysis buffer (PBS containing 2% Triton X-100, 1 mg ml −1 lysozyme and protease inhibitors). After freeze-thawing, bacteria were sonicated on ice and centrifuged at 18,000 g for 30 min at 4 °C. Supernatants were purified on prepacked fast-flow Gluthathione Sepahrose 4B columns (Sigma) according to the manufacturer’s instructions. Flag-tagged proteins were expressed in HEK cells and purified by incubating cell lysate with FLAG-sepharose beads (Sigma) according to the manufacturer’s instructions. One microgram of purified GST-Nck1 or GST was immobilized on GSH beads and incubated with 1 μg of purified FLAG-c-Cbl and increasing amounts (0, 0.25, 0.5 or 1 μg) of FLAG-Synpo-T. Proteins were analysed using SDS–PAGE and western blotting. Immunocytochemistry For immunocytochemistry, podocytes were fixed with 2% paraformaldehyde and 4% sucrose in PBS for 5 min followed by permeabilization with 0.3 % Triton X-100 in PBS for 5 min at room temperature. After rinsing with PBS, unspecific binding sites were blocked with 2% FCS, 2% BSA and 0.2 % fish gelatine in PBS for 30 min. Filamentous actin was decorated with rhodamine-labelled phalloidin (Molecular Probes) at 1:750 in PBS for 30 min to visualize stress fibres [13] . To visualize ARP3 (ref. 27 ), a rabbit polyclonal anti-ARP3 (Millipore) was used at 1:50, followed by Alexa Flour 488-conjugated anti-rabbit IgG (Molecular Probes) at 1:700. Confocal images were acquired with a Zeiss upright confocal microscope. Images from an optical slice of ~1–5 μm were acquired at a resolution of 1,200 pixels per inch with the Zeiss Pascal software [33] . Image analysis was performed in ImageJ or Adobe Photoshop for Mac OS X. Stress fibre quantification A stress fibre was defined as a phalloidin-positive structure that was represented by a line spanning the length of the cell. ‘Broken’ lines and ‘arcs’ were not counted as stress fibres [33] . We counted stress fibres manually in each individual cell in independent images. We included at least three independent trials for each experimental condition, where >50 cells were counted in each trial in 5–10 independent images per trial. Statistical analysis Statistical significance was evaluated using the GraphPad Prism 6.0 software by one-way ANOVA with Dunenett’s multiple comparison test when multiple groups were analysed. For the comparison of two groups Student’s t -test was applied. P <0.05 was considered significant. Values are reported as mean±s.e.m. How to cite this article: Buvall, L. et al. Proteasomal degradation of Nck1 but not Nck2 regulates RhoA activation and actin dynamics. Nat. Commun. 4:2863 doi: 10.1038/ncomms3863 (2013).